A C2 domain protein kinase initiates phagocytosis in the protozoan parasiteEntamoeba histolytica Phagocytosis is a process whereby particles are taken in by cells through mechanisms superficially similar to those for endocytosis. It serves a wide range of functions, from providing nutrition in unicellular organisms to initiation of both innate and adaptive immunity in vertebrates. In the protozoan parasite Entamoeba histolytica , it has an essential role in survival and pathogenesis. In this study, we show that EhC2PK, a C2-domain-containing protein kinase, and the Ca 2+ and actin-binding protein, EhCaBP1, are involved in the initiation of phagocytosis in E. histolytica . Conditional suppression of EhC2PK expression and overexpression of a mutant form reveals its role in the initiation of phagocytic cups. EhC2PK binds phosphatidylserine in the presence of Ca 2+ and thereby recruits EhCaBP1 and actin to the membrane. Identification of these proteins in phagocytosis is an important step in amoebic biology and these molecules could be the important targets for developing novel therapies against amoebiasis. Phagocytosis has a critical role in the biology and pathogenesis of the protozoan parasite Entamoeba histolytica . Trophozoites partly source their nutrients by phagocytosis of bacterial and other cells found in the intestine. The trophozoites then digest the cells and re-utilize the nutrients [1] , [2] . Erythrophagocytosis is a pathogenic marker of amoebiasis and it occurs frequently during invasive disease [3] . Phagocytosis of dead epithelial, immune and nonimmune cells is also thought to be one of the important features of amoebic pathogenesis [4] , [5] . So far no defined receptor(s) or ligand(s) that initiate phagocytosis in E. histolytica have been identified. Although there is some evidence to suggest that Gal/GalNAc lectin is likely to be one of the phagocytosis receptors, engagement of the lectin does not always lead to phagocytosis [6] , [7] . In mammalian cells, the most studied phagocytic system is Fc receptor-mediated phagocytosis. The process is initiated when FcR on the surface of a phagocyte binds to immunoglobulin-coated opsonized particles. At sites of phagocytosis, the plasma membrane is pulled around the target particles leading to the formation of phagocytic cups [8] . This is followed by constriction at the distal margins of the cup that results in closure of the phagosome. Transient assembly of actin filaments and myosin-dependent contractile activities have critical roles in different steps of this process [9] . Initiation of phagocytosis is achieved by ligand-induced Fcγ receptor clustering that leads to the activation of membrane associated Src family of kinases [10] that phosphorylate the immune-receptor tyrosine-based activation motif of FcR, which in turn recruits the syk family of tyrosine kinases [11] . syk kinase phosphorylates PI3K resulting in the presence of PI3K close to the clustered FcR region of the membrane [12] . A nonphagocytic cell can be induced to initiate phagocytosis by expression of FcR and syk , suggesting that syk has an important role in phagocytic signal transduction from FcR [7] . In the presence of PI3K inhibitors, incomplete phagosomes appear as actin-rich phagocytic cups, suggesting that PI3K may be involved in organizing the later stages of phagocytosis [13] , [14] , [15] . Ca 2+ signals are generated subsequent to the activation of FcγR through downstream processes that involve activation of PLCγ and are required for phagosome closure and maturation mainly through actin remodeling [16] . It is not clear whether Ca 2+ signalling has any role in the process of initiation. A number of molecules have been implicated to participate in amoebic phagocytosis, although many of the known players of the mammalian system have not been identified in this organism. Therefore, phagocytosis in E. histolytica is likely to follow a different molecular path. Some of the molecules that have been identified are components of the cytoskeleton [17] and its regulators [18] , [19] , [20] , [21] , [22] , [23] , [24] , [25] including phosphoinositides and one of the FYVE-domain-containing protein EhFP4 [26] . Analysis of the phagosome proteome has revealed involvement of a large number of proteins in phagosome formation and subsequent maturation [27] , [28] . The list includes novel proteins, such as phagosome-associated transmembrane kinase and the serine-rich E. histolytica protein [29] . Cytoplasmic Ca 2+ is known to be involved in the process of phagocytosis. However, no mechanistic details about the process of initiation or the involvement of Ca 2+ are available. Although much progress has been made in deciphering the pathways leading to phagocytosis in different organisms including E. histolytica , the early events of the process remain to be discovered. Our previous studies have shown the involvement of E. histolytica calcium-binding protein (EhCaBP1) in actin dynamics. Downregulation of this protein leads to defects in both phagocytosis and pseudopod formation [30] . EhCaBP1 binds both G- and F-actin in vitro and in vivo . The absence of this molecule in the phagosome and its rapid recruitment at the site of phagocytosis (total time from its appearance to its eventual disappearance spans about 30–40 s) suggests that EhCaBP1 may be involved in events just subsequent to the attachment of ligand particles [31] . To explore the events just before the appearance of EhCaBP1 at the phagocytosis site, we decided to look for the proteins that bind to EhCaBP1 and test their involvement in phagocytosis. EhC2PK, a novel C2-domain-containing protein kinase, was identified as an EhCaBP1-binding protein. In this report, we show that EhC2PK along with EhCaBP1 is required for the initiation of phagocytosis in E. histolytica . We have used both antisense and dominant negative approaches for functional dissection. Our results indicate that erythrophagocytosis is initiated by the recruitment of EhC2PK at the site of red blood cell (RBC) attachment and then subsequently the recruitment of EhCaBP1 and actin. We are also able to distinguish steps that require Ca 2+ from those that do not. Thus, identification of these proteins involved in parasite phagocytosis may provide targets for therapeutic intervention in parasite-mediated disease. Identification of EhC2PK as an EhCaBP1-binding protein Affinity chromatography using EhCaBP1-Sepharose columns resulted in elution of a number of proteins that bound to EhCaBP1 as described before [32] . The bound proteins were identified by mass spectrometric analysis ( Supplementary Table S1 ). The binding proteins included actin, a known binding partner of EhCaBP1, and a C2-domain-containing protein kinase (EhC2PK), which was selected for further study ( Fig. 1a ). EhC2PK differs from typical PKCs with respect to the absence of a C1 domain, which is necessary for the interaction with diacylglycerol. Sequence similarity searches using the kinase domain of EhC2PK showed maximum identity (45%) with Ca 2+ /CaM-dependent protein kinases of humans, but not with other C2-domain-containing kinases. We conclude from these observations that EhC2PK is distinctly different from other C2-domain-containing protein kinases, including PKC. 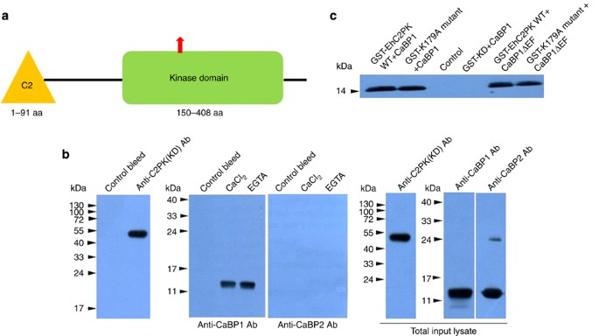Figure 1: EhCaBP1 binds EhC2PKin vitroandin vivo. (a) Schematic presentation of domain organization of EhC2PK. The protein has a molecular mass of 50 kDa and two domains, C2 (1–91 amino-acid residues) and protein kinase (150–408 amino-acid residues). The active site of the kinase was predicted to reside within 269–281 amino-acid residues (arrow). (b) Immunoprecipitation of EhCaBP1 from whole-cell lysate ofE. histolyticausing CNBr-conjugated anti-C2PK antibody. EhC2PK was also immunoprecipitated from the lysate using CNBr-conjugated anti-C2PK antibody as a control. The total input lysate was also probed for the presence of EhC2PK, EhCaBP1 and EhCaBP2 by their respective antibodies. (c) Co-precipitation of EhCaBP1 or its calcium-binding defective mutant EhCaBP1ΔEF with wild-type GST-EhC2PK and GST-K179A mutant.In vitroGST-tagged kinase domain alone (GST-KD) was not able to precipitate EhCaBP1. GST alone did not bind to EhCaBP1. Glutathione Sepharose beads were used for precipitation experiments. All molecular markers are in kDa. Figure 1: EhCaBP1 binds EhC2PK in vitro and in vivo . ( a ) Schematic presentation of domain organization of EhC2PK. The protein has a molecular mass of 50 kDa and two domains, C2 (1–91 amino-acid residues) and protein kinase (150–408 amino-acid residues). The active site of the kinase was predicted to reside within 269–281 amino-acid residues (arrow). ( b ) Immunoprecipitation of EhCaBP1 from whole-cell lysate of E. histolytica using CNBr-conjugated anti-C2PK antibody. EhC2PK was also immunoprecipitated from the lysate using CNBr-conjugated anti-C2PK antibody as a control. The total input lysate was also probed for the presence of EhC2PK, EhCaBP1 and EhCaBP2 by their respective antibodies. ( c ) Co-precipitation of EhCaBP1 or its calcium-binding defective mutant EhCaBP1ΔEF with wild-type GST-EhC2PK and GST-K179A mutant. In vitro GST-tagged kinase domain alone (GST-KD) was not able to precipitate EhCaBP1. GST alone did not bind to EhCaBP1. Glutathione Sepharose beads were used for precipitation experiments. All molecular markers are in kDa. Full size image We confirmed binding of the two proteins by immunoprecipitation using an immobilized anti-EhC2PK antibody and the total cell lysate of E. histolytica trophozoites. EhC2PK antibody precipitated not only EhC2PK, but also EhCaBP1 from the total cell lysate ( Fig. 1b ). EGTA did not affect the interaction between the two molecules. This interaction is highly specific as EhCaBP2, a protein with high sequence similarity with EhCaBP1 (79% identity at the amino-acid level) but with a different function [33] , was not detected in the immunoprecipitate. Our data show that the EhC2PK and EhCaBP1 interaction does not require Ca 2+ in spite of both proteins being calcium-binding proteins. To demonstrate the interaction of EhC2PK with EhCaBP1 in vitro , we expressed EhC2PK as a GST-tagged protein and incubated it with EhCaBP1. The protein complex was obtained by binding to glutathione-Sepharose and EhCaBP1 was detected using a specific antibody by western blotting ( Fig. 1c ). There was no nonspecific binding of EhCaBP1 to the beads as no signal was detected in the lane containing glutathione- S -transferase (GST) alone. We checked whether an intact kinase domain is required for this binding by carrying out an in vitro binding assay using GST-tagged wild-type (WT) EhC2PK, a kinase-dead mutant (K179A) and the kinase domain alone ( Fig. 1c ). The kinase domain alone is functionally active as it can autophosphorylate as well as phosphorylate external substrates, such as histone and myelin basic protein. The K179A mutant did not show any kinase activity. Both the WT and kinase-dead mutant bound EhCaBP1, but the kinase domain alone could not bind to EhCaBP1 (GST-KD; Fig. 1c ). A mutant form of EhCaBP1 (CaBP1ΔEF), which is defective in Ca 2+ -binding [31] , was also able to bind WT and the K179A mutant of EhC2PK. Taken together, these experiments indicate that EhCaBP1 is an interacting partner of EhC2PK and that binding does not require the kinase domain or Ca 2+ . The C2 domain may be involved in this binding; however, we could not test the direct interaction of the C2 domain with EhCaBP1, as the C2 domain was insoluble under binding conditions. EhC2PK binds phosphatidylserine and recruits EhCaBP1 and actin C2 domains generally display the property of Ca 2+ -dependent lipid binding. When compared with all known C2 domains, that of EhC2PK shows a maximum identity of 30% with C2 domains of Ca 2+ -dependent PKCβ and -γ of Homo sapiens ( Supplementary Fig. S1 ). However, it is smaller in length compared with other C2 domains, including the C2 domain of amoebic protein EhC2A. As the C2 domain of EhC2PK is somewhat different from other C2 domains, we tested the ability of the C2 domain of EhC2PK to bind Ca 2+ using a 45 Ca 2+ overlay assay ( Supplementary Fig. S2 ). The binding of radioactive Ca 2+ to the purified C2 domain band in the blot confirmed the ability of this protein to bind Ca 2+ . As EhCaBP1 binds to EhC2PK, it is possible that it is recruited to the plasma membrane through binding to EhC2PK. To test this we first checked the ability of EhC2PK and then both EhC2PK and EhCaBP1 to bind phospholipid liposomes in the presence and absence of Ca 2+ . We mixed the liposomes with the indicated proteins and the binding was assessed by sedimentation and western blotting. The sedimentation of EhC2PK along with liposomes, in the presence of Ca 2+ but not EGTA, suggested that EhC2PK binds phosphatidylserine in a Ca 2+ -dependent manner ( Fig. 2a ). We did not observe any binding when the kinase domain alone was used in the liposome sedimentation assay ( Fig. 2b ). We could not test the ability of the C2 domain to bind lipids and EhCaBP1 because of the insoluble nature of C2 peptide as mentioned previously. We did not observe binding of EhCaBP1 to the liposomes in the presence of Ca 2+ or EGTA ( Fig. 2c ). GST was used as a control to show that the tag by itself did not bind to liposomes ( Fig. 2c ). We incubated liposomes with EhC2PK and EhCaBP1 together and found both the proteins in the pellet fraction in the presence of Ca 2+ , suggesting that EhCaBP1 can bind to liposomes only through EhC2PK and this required Ca 2+ ( Fig. 2a ). We investigated the specificity of the interaction between EhC2PK and phospholipids using phosphatidylcholine (PC) instead of phosphatidylserine. We did not observe any protein in the pellet, suggesting that EhC2PK preferentially binds phosphatidylserine. The GST-tagged full-length protein did not bind to PC liposomes either in the presence or in the absence of Ca 2+ as all the protein was found in supernatant ( Fig. 2d ). The purified kinase domain alone also did not bind to liposomes ( Fig. 2e ). Furthermore, GST and EhCaBP1 did not bind PC-containing liposomes in the presence of Ca 2+ , as none of the proteins were present in the liposome pellet ( Fig. 2f,g ). These findings are consistent with the properties of other C2-domain-containing proteins, in which binding to phosphatidylserine is mediated through the C2 domain [34] , [35] . We conclude from these results that EhCaBP1 binds lipids through EhC2PK and this interaction is lipid-specific and requires the presence of Ca 2+ . Further, we carried out experiments to investigate whether liposomes-containing EhC2PK and EhCaBP1 are able to bind to actin filaments. We observed that liposomes incubated with EhC2PK and EhCaBP1 could bind to actin filaments in a Ca 2+ -dependent manner, whereas liposomes incubated with just EhCaBP1 or EhC2PK could not ( Supplementary Fig. S3 ). 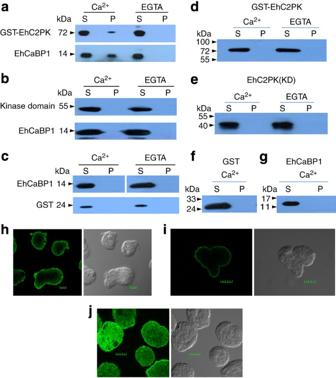Figure 2: EhC2PK binds phosphatidylserine in the presence of Ca2+. Presence of specific proteins in the pellet (P), that is, liposome fraction indicates binding. Proteins that do not bind remain in the soluble fraction (S). (a) Purified GST-EhC2PK and EhCaBP1 were incubated with phosphatidylserine (PS) liposomes in the presence and the absence of Ca2+. (b) Recombinant His-tagged kinase domain was incubated with PS liposomes in the presence of Ca2+and EGTA. (c) EhCaBP1 and GST were incubated with PS liposomes in the presence or the absence of Ca2+. (d) Purified GST-EhC2PK was incubated with phosphatidylcholine (PC) liposomes in the presence and the absence of Ca2+. (e) Purified kinase domain was also incubated with PC liposomes in the presence of Ca2+and EGTA. (f,g) GST and EhCaBP1 were also incubated with PC liposomes in the presence Ca2+. Immunoblot analysis was carried out using anti-GST and anti-EhCaBP1 antibodies. (h) Localization of EhC2PK in normal cells. (i) EhC2PK localization after cells were treated with ionomycin for 15 min and (j) in the presence of BAPTA-AM for 15 min. The EhC2PK was stained by anti-EhC2PK antibody followed by Alexa 488-labelled second antibody (scale bar, 10 μm). Figure 2: EhC2PK binds phosphatidylserine in the presence of Ca 2+ . Presence of specific proteins in the pellet (P), that is, liposome fraction indicates binding. Proteins that do not bind remain in the soluble fraction (S). ( a ) Purified GST-EhC2PK and EhCaBP1 were incubated with phosphatidylserine (PS) liposomes in the presence and the absence of Ca 2+ . ( b ) Recombinant His-tagged kinase domain was incubated with PS liposomes in the presence of Ca 2+ and EGTA. ( c ) EhCaBP1 and GST were incubated with PS liposomes in the presence or the absence of Ca 2+ . ( d ) Purified GST-EhC2PK was incubated with phosphatidylcholine (PC) liposomes in the presence and the absence of Ca 2+ . ( e ) Purified kinase domain was also incubated with PC liposomes in the presence of Ca 2+ and EGTA. ( f , g ) GST and EhCaBP1 were also incubated with PC liposomes in the presence Ca 2+ . Immunoblot analysis was carried out using anti-GST and anti-EhCaBP1 antibodies. ( h ) Localization of EhC2PK in normal cells. ( i ) EhC2PK localization after cells were treated with ionomycin for 15 min and ( j ) in the presence of BAPTA-AM for 15 min. The EhC2PK was stained by anti-EhC2PK antibody followed by Alexa 488-labelled second antibody (scale bar, 10 μm). Full size image We extended our studies to investigate the role of Ca 2+ in the membrane localization of EhC2PK using immunofluorescence. In amoebic cells, the majority of stained EhC2PK is found near the plasma membrane with some amount in the cytoplasm ( Fig. 2h ). When we treated the cells with the ionophore ionomycin, almost all of the fluorescence was located at the plasma membrane ( Fig. 2i ). However, when we depleted the free cytoplasmic Ca 2+ with BAPTA-AM, only cytoplasmic fluorescence was observed ( Fig. 2j ). These results support our in vitro observations regarding the requirement of Ca 2+ in membrane localization of EhC2PK. The results of this study together with our earlier observations regarding the ability of a mutant protein, CaBP1ΔEF, which is defective in binding Ca 2+ in recruitment to the phagocytic cups [31] , suggests that Ca 2+ is required for membrane localization of EhC2PK but not for its binding to EhCaBP1. The C2 domain is involved in membrane localization of EhC2PK To check whether the C2 or the kinase domain is involved in lipid binding and membrane localization, we checked the ability of the domains to bind lipids or membranes in vivo . Membrane binding in cells was checked by expressing individual domains of the protein in E. histolytica cells as GFP tags ( Fig. 3a ). We first showed that the GFP tag did not alter the property of the EhC2PK, as we observed similar distribution of immunostained EhC2PK and EhC2PK-GFP in amoebic cells ( Fig. 3b,c ). Green fluorescent stains of EhC2PK-GFP were clearly visible on phagocytic cups and these colocalized with actin. The distributions of KD-GFP and C2-GFP were also observed in their respective cell lines ( Fig. 3d,e ). Although KD-GFP was mainly seen in the cytoplasm, C2-GFP was essentially found at the membrane, consistent with our results from in vitro studies. Hence, the membrane localization of EhC2PK is determined by the C2 domain of the protein. 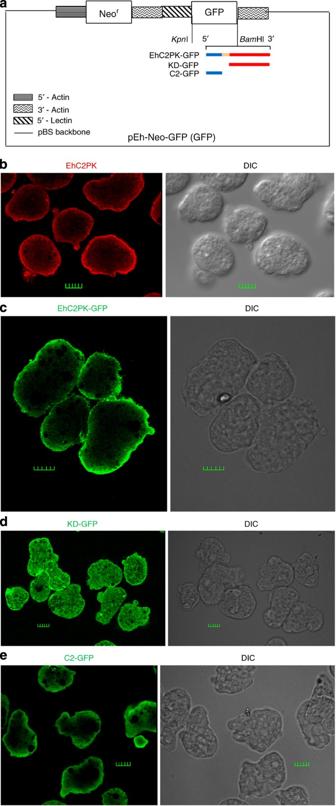Figure 3: C2 domains are required for membrane localization of EhC2PK. (a) Schematic representation of the proteins expressed in constitutive expression system as GFP-conjugated proteins. Immunolocalization of: (b) EhC2PK in normal cells (without any constructs), (c) GFP-tagged EhC2PK (EhC2PK-GFP) in cells carrying the tagged construct, (d) GFP-tagged kinase domain (KD-GFP) in cells carrying KD-GFP construct and (e) GFP-tagged C2 domain (C2-GFP) in cells carrying this construct are shown. The wild-type EhC2PK was labelled by Alexa 546 and GFP-tagged proteins were visualized by anti-GFP antibody followed by Alexa 488-labelled secondary antibody (scale bar, 10 μm; DIC, differential interference contrast). Figure 3: C2 domains are required for membrane localization of EhC2PK. ( a ) Schematic representation of the proteins expressed in constitutive expression system as GFP-conjugated proteins. Immunolocalization of: ( b ) EhC2PK in normal cells (without any constructs), ( c ) GFP-tagged EhC2PK (EhC2PK-GFP) in cells carrying the tagged construct, ( d ) GFP-tagged kinase domain (KD-GFP) in cells carrying KD-GFP construct and ( e ) GFP-tagged C2 domain (C2-GFP) in cells carrying this construct are shown. The wild-type EhC2PK was labelled by Alexa 546 and GFP-tagged proteins were visualized by anti-GFP antibody followed by Alexa 488-labelled secondary antibody (scale bar, 10 μm; DIC, differential interference contrast). Full size image EhC2PK is involved in erythrophagocytosis We generated conditional EhC2PK knockdown cells ( Fig. 4a ) using tetracycline inducible antisense expression, as previously described [30] . Overexpression of antisense EhC2PK RNA in the presence of tetracycline specifically reduced the level of EhC2PK by about 70% without affecting the levels of EhCaBP1 ( Fig. 4b ). We also generated cells that overexpress EhC2PK ( Fig. 4c ) and the K179A mutant by cloning the gene in the sense orientation in the tetracycline inducible vector system. Erythrophagocytosis in these cell lines was measured in the presence and absence of tetracycline. We observed 68 and 50% reduction in erythrophagocytosis by cells expressing the antisense gene and K179A mutant, respectively, compared with the cells containing vector alone ( Fig. 4d ). Cells with the gene in the sense orientation and grown in the presence of tetracycline and cells with the gene in antisense orientation grown in the absence of tetracycline showed similar levels of phagocytosis ( Fig. 4d ). To further understand the involvement of EhC2PK in erythrophagocytosis we carried out immunostaining; EhC2PK was found at the phagocytic cups along with EhCaBP1 and actin ( Fig. 4e,f ). The enrichment of these molecules at the phagocytic cups was quantified by determining the amount of stain in phagocytic cups compared with the staining intensity of the other regions of the membrane. We did not observe EhC2PK in newly formed phagosomes ( Fig. 4g ), nor did we see any phagocytic cup formation in the antisense cell lines (EhC2PK AS), although a number of RBCs were attached to the membrane ( Fig. 4h ). As a control for membrane staining, we used the membrane protein EhTMK-9 that uniformly stains the plasma membrane of E. histolytica [36] ( Fig. 5a ). EhTMK-9 is also found in newly formed phagosomes and along with actin that can be used as a marker for phagosomes. Quantitative analysis of specific immunostaining showed a significantly higher level of EhC2PK in the phagocytic cups compared with other parts of the membrane ( Fig. 5b ). EhTMK-9 stained both the phagocytic cups and the rest of the plasma membrane equally ( Fig. 5b ). There was no significant difference in the intensity of EhTMK-9 in the nonphagocytic part of the membrane and in phagocytic cups. However, there was a significant increase in the EhC2PK stain in phagocytic cups compared with any other parts of the membrane. Quantitative analysis of the specific immunostains showed the presence of EhTMK-9 and the lack of EhC2PK in the phagosomes ( Fig. 5c ). Similar analysis with EhCaBP1 antibody also showed significant enrichment of EhCaBP1 in phagocytic cups but not in phagosomes ( Supplementary Fig. S4 ). 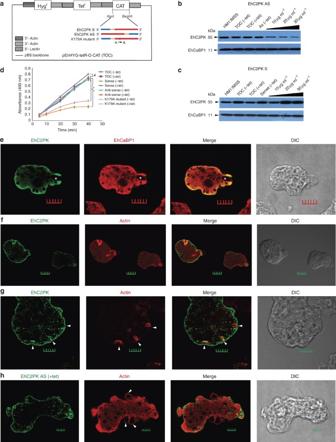Figure 4: EhC2PK is involved in initiation of phagocytosis. (a) Schematic representation of different constructs of pEhHYG-tetR-O-CAT (tetracycline inducible) vector used in the study. (b,c) Immunoblot analysis of amoebic cells with indicated recombinant constructs ('AS'-antisense, 'S'-sense) in the presence and the absence of tetracycline. (d) Erythrocyte uptake performed with cell lines as indicated in the presence and the absence of tetracycline. The experiment was repeated three times independently in triplicates (N=3 with error bars indicating the standard error). The statistical comparisons were made by one-way ANOVA test.P-values for * and ** are P<0.01 andP<0.001, respectively.#P>0.05. (e)E. histolyticacells undergoing erythrophagocytosis were stained for EhC2PK and EhCaBP1, the phagocytic cup is marked by an asterisk. The cells were double labelled with Alexa 488 (EhC2PK) and Alexa 546 (EhCaBP1). (f) Cells actively erythrophagocytosing were stained for EhC2PK and actin. (g)E. histolyticacells stained for EhC2PK and actin, the newly formed phagosome and phagocytic cups are marked by arrow. (h) Cells overexpressing antisense RNA were incubated with RBCs. The cells were double labelled with Alexa 488 (EhC2PK) and TRITC-Phalloidin (actin) (scale bar, 10 μm; DIC, differential interference contrast). Figure 4: EhC2PK is involved in initiation of phagocytosis. ( a ) Schematic representation of different constructs of pEhHYG-tetR-O-CAT (tetracycline inducible) vector used in the study. ( b , c ) Immunoblot analysis of amoebic cells with indicated recombinant constructs ('AS'-antisense, 'S'-sense) in the presence and the absence of tetracycline. ( d ) Erythrocyte uptake performed with cell lines as indicated in the presence and the absence of tetracycline. The experiment was repeated three times independently in triplicates ( N =3 with error bars indicating the standard error). The statistical comparisons were made by one-way ANOVA test. P -values for * and ** are P<0.01 and P <0.001, respectively. # P >0.05. ( e ) E. histolytica cells undergoing erythrophagocytosis were stained for EhC2PK and EhCaBP1, the phagocytic cup is marked by an asterisk. The cells were double labelled with Alexa 488 (EhC2PK) and Alexa 546 (EhCaBP1). ( f ) Cells actively erythrophagocytosing were stained for EhC2PK and actin. ( g ) E. histolytica cells stained for EhC2PK and actin, the newly formed phagosome and phagocytic cups are marked by arrow. ( h ) Cells overexpressing antisense RNA were incubated with RBCs. The cells were double labelled with Alexa 488 (EhC2PK) and TRITC-Phalloidin (actin) (scale bar, 10 μm; DIC, differential interference contrast). 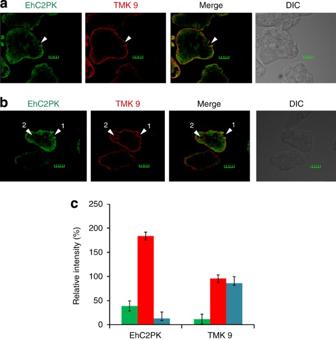Figure 5: Localization of EhC2PK and pan membrane protein EhTMKB1-9 in cells undergoing erythrophagocytosis. (a) Amoebic cells undergoing erythrophagocytosis stained for EhC2PK and TMK-9 (phagocytic cup marked by arrow). (b) A newly formed phagocytic cup (marked 1) and a phagosome (marked 2). (c) Intensity of immunostain (EhC2PK, EhTMK-9) was measured at multiple locations in the membrane and average relative intensity was computed by taking the signal from membrane as 100% for each marker separately. Quantitative estimation of immunostained signals in phagosomes compared with the phagocytic cups and the cytoplasm is shown. EhC2PK and TMK-9 are stained by Alexa488 and Alexa546, respectively (green, cytosol; red, phagocytic cups; blue, phagosome). Forc, five random regions were selected from membrane, cytosol and phagocytic cups and average intensity was computed for each region. This was repeated for four such cells (N=4, bars represent standard error; scale bar, 10 μm ; DIC, differential interference contrast). Full size image Figure 5: Localization of EhC2PK and pan membrane protein EhTMKB1-9 in cells undergoing erythrophagocytosis. ( a ) Amoebic cells undergoing erythrophagocytosis stained for EhC2PK and TMK-9 (phagocytic cup marked by arrow). ( b ) A newly formed phagocytic cup (marked 1) and a phagosome (marked 2). ( c ) Intensity of immunostain (EhC2PK, EhTMK-9) was measured at multiple locations in the membrane and average relative intensity was computed by taking the signal from membrane as 100% for each marker separately. Quantitative estimation of immunostained signals in phagosomes compared with the phagocytic cups and the cytoplasm is shown. EhC2PK and TMK-9 are stained by Alexa488 and Alexa546, respectively (green, cytosol; red, phagocytic cups; blue, phagosome). For c , five random regions were selected from membrane, cytosol and phagocytic cups and average intensity was computed for each region. This was repeated for four such cells ( N =4, bars represent standard error; scale bar, 10 μm ; DIC, differential interference contrast). Full size image In general, proteins that are known to be involved in phagocytosis are found in phagosomes [27] . In previous studies, the phagosome proteome was investigated to identify proteins that may be involved in phagocytosis. Although many known proteins involved in phagocytosis were found in the proteome, neither EhC2PK nor EhCaBP1 was among the list of proteins in two different studies [28] , [29] . The absence of both EhC2PK and EhCaBP1 in phagosomes, suggests that these may be exclusively associated with the early steps of phagocytosis. We next determined whether the process of phagocytosis is delayed in the antisense cell line by observing cup formation at different times after addition of RBCs. At 3 min, there was no initiation of phagocytosis in these cells or in cells containing the C2 domain alone or the K179A mutant ( Fig. 6a ). However, on longer incubation (5 and 8 min), initiation was observed in these cell lines, suggesting that the rate of initiation has slowed down ( Fig. 6a,b ). We also measured the ability of these overexpressing cell lines to take up RBCs. Overexpression of the full-length protein resulted in an enhanced level of erythrophagocytosis. Reduction of uptake was observed only when the C2 domain was overexpressed, thereby displaying a dominant negative phenotype ( Fig. 6c ). We did not observe any significant difference in the rate of phagocytosis in cells overexpressing the kinase domain. Although kinase domain overexpression did not give a dominant negative phenotype, its functional involvement was evident in the cell lines induced to overexpress the kinase-dead mutant ( Fig. 4d ). These results indicate that EhC2PK, similar to EhCaBP1, is also involved in the process of erythrophagocytosis and that these proteins are essential for the process of initiation of phagocytosis. C2-GFP and EhC2PK (K179A) were observed to be enriched in phagocytic cups along with EhCaBP1 after 8 min of incubation in cells overexpressing these proteins ( Fig. 6d,e ). The overexpression of mutant proteins delayed the rate of erythrophagocytosis by competing with the endogenous WT protein. This result indicates that the C2 domain alone is sufficient for recruiting EhCaBP1 to phagocytic cups. 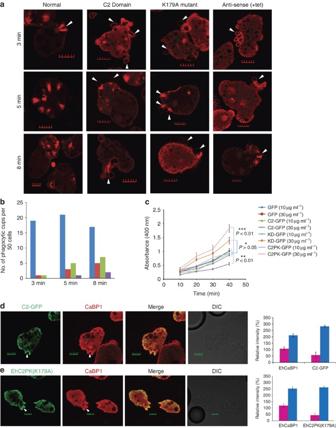Figure 6: EhC2PK is essential for initiation of phagocytosis. (a) Cells with and without mentioned constructs were incubated with human erythrocytes for indicated time points and then were fixed and stained with TRITC-Phalloidin. Initiation of phagocytosis was marked by accumulation of actin at the phagocytic cups (marked by an arrow). (b) Fifty cells were randomly selected for each experiment and the number of phagocytic cups present in all the cells were enumerated (blue, normal HM1:MSS; red, C2-domain; green, K179A mutant; purple, antisense). (c) Erythrocyte uptake was determined quantitatively using RBC solubilization assay. The level of expression of cloning indicated that the gene was manipulated by using two different concentrations of G418 (10 and 30 μg ml−1). The experiment was repeated five times independently in triplicates (N=5) with error bars indicating the standard error. The statistical comparisons were carried out using one-way ANOVA test. 'P-values' are mentioned in the figure (theP>0.05 for KD-GFP at 30 μg ml−1, which implies that RBC uptake was not significantly higher than other cell lines maintained at 10 μg ml−1of G418). (d) Localization of C2-GFP and EhCaBP1 in C2-GFP-expressing cells after 8 min of incubation with RBC. Quantitative analysis of the fluorescent signals of cells undergoing erythrophagocytosis and expressing C2-GFP and EhCaBP1 are shown (pink, cytosol; blue, phagocytic cups). (e) Localization of EhCaBP1 in K179A mutant expressing cells after 8 min of incubation with RBC (pink, cytosol; blue, phagocytic cups). For analysis, five random regions were selected from membrane, cytosol and phagocytic cups and average intensity was computed for each region. This was repeated for four such cells (N=4, bars represent standard error). Relative intensity was calculated by assuming intensity from membrane as 100% for each marker separately (scale bar, 10 μm; DIC, differential interference contrast). Figure 6: EhC2PK is essential for initiation of phagocytosis. ( a ) Cells with and without mentioned constructs were incubated with human erythrocytes for indicated time points and then were fixed and stained with TRITC-Phalloidin. Initiation of phagocytosis was marked by accumulation of actin at the phagocytic cups (marked by an arrow). ( b ) Fifty cells were randomly selected for each experiment and the number of phagocytic cups present in all the cells were enumerated (blue, normal HM1:MSS; red, C2-domain; green, K179A mutant; purple, antisense). ( c ) Erythrocyte uptake was determined quantitatively using RBC solubilization assay. The level of expression of cloning indicated that the gene was manipulated by using two different concentrations of G418 (10 and 30 μg ml −1 ). The experiment was repeated five times independently in triplicates ( N =5) with error bars indicating the standard error. The statistical comparisons were carried out using one-way ANOVA test. ' P -values' are mentioned in the figure (the P >0.05 for KD-GFP at 30 μg ml −1 , which implies that RBC uptake was not significantly higher than other cell lines maintained at 10 μg ml −1 of G418). ( d ) Localization of C2-GFP and EhCaBP1 in C2-GFP-expressing cells after 8 min of incubation with RBC. Quantitative analysis of the fluorescent signals of cells undergoing erythrophagocytosis and expressing C2-GFP and EhCaBP1 are shown (pink, cytosol; blue, phagocytic cups). ( e ) Localization of EhCaBP1 in K179A mutant expressing cells after 8 min of incubation with RBC (pink, cytosol; blue, phagocytic cups). For analysis, five random regions were selected from membrane, cytosol and phagocytic cups and average intensity was computed for each region. This was repeated for four such cells ( N =4, bars represent standard error). Relative intensity was calculated by assuming intensity from membrane as 100% for each marker separately (scale bar, 10 μm; DIC, differential interference contrast). Full size image To distinguish between recruitment and subsequent signal transduction processes we carried out colocalization experiments with C2-GFP, the kinase-dead mutant of EhC2PK-GFP, EhCaBP1 and actin during erythrophagocytosis and pseudopod formation. Pairwise analysis of these proteins clearly showed that the C2 domain alone could colocalize with EhCaBP1 and actin ( Fig. 7 ). We also found enrichment of EhCaBP1 at the phagocytic cups in cells overexpressing the kinase-dead mutant of EhC2PK. Therefore, it seems that the recruitment process does not require the kinase domain, but it is necessary in subsequent steps. The interaction of a C2-domain-containing kinase with a multi-EF hand Ca 2+ -binding protein is unique, as no such examples are known from any other system. 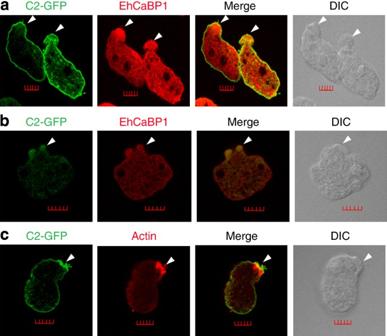Figure 7: C2 domain colocalizes with EhCaBP1 and actin. (a) Cells expressing C2-GFP at low level show enrichment of C2 domain at pseudopods along with EhCaBP1 (shown by arrow). (b) C2-GFP colocalizes with EhCaBP1 in cells undergoing erythrophagocytosis as shown by arrow. (c) C2-GFP shows enrichment at the site of initiation of phagocytosis, which is marked by accumulation of actin. The C2-GFP is probed by anti-GFP antibody and Alexa488-labelled secondary antibody. The actin is stained by TRITC-Phalloidin and EhCaBP1 by Alexa546. All cells were maintained at 10 μg ml−1G418 during the experiment (scale bar, 10 μm; DIC, differential interference contrast). Figure 7: C2 domain colocalizes with EhCaBP1 and actin. ( a ) Cells expressing C2-GFP at low level show enrichment of C2 domain at pseudopods along with EhCaBP1 (shown by arrow). ( b ) C2-GFP colocalizes with EhCaBP1 in cells undergoing erythrophagocytosis as shown by arrow. ( c ) C2-GFP shows enrichment at the site of initiation of phagocytosis, which is marked by accumulation of actin. The C2-GFP is probed by anti-GFP antibody and Alexa488-labelled secondary antibody. The actin is stained by TRITC-Phalloidin and EhCaBP1 by Alexa546. All cells were maintained at 10 μg ml −1 G418 during the experiment (scale bar, 10 μm; DIC, differential interference contrast). Full size image In this study, we show the involvement of two novel molecules, EhC2PK and EhCaBP1, in the initiation of erythrophagocytosis in E. histolytica . Phagocytosis is a fundamental process in a variety of cell types and involves initiation and subsequent closure and maturation of the phagosome. The best-studied system is the phagocytosis of opsonized bacteria through immunoglobulin Fc receptors. Here, the process is initiated by the occupancy of receptors and their clustering, which leads to activation of a protein kinase, such as syk [11] . Receptor activation also stimulates class I PI3K through phosphorylation of the p85 regulatory subunit. This causes production of PtdIns(3,4,5)P 3 beneath the phagocytic cups, and activation of PLC and PLD. Ca 2+ is released, which mobilizes InsP 3 [12] . Therefore, Ca 2+ is thought to have a major role in phagosome closure and maturation, mainly due to the process of actin remodeling [35] , [36] . The mechanism of initiation of phagocytosis is not clear and many of the participating molecules have not yet been identified. This is particularly so in protozoa. In E. histolytica , it has not been possible to study initiation as a distinct process separate from closure and maturation, partly due to the short duration of the process and the lack of information regarding phagocytic receptors on the cell surface of E . histolytica . Here, we have delineated the initial steps in the phagocytic process. The first step in which Ca 2+ is required is the recruitment of EhC2PK at the RBC attachment sites. In the absence of Ca 2+ , most of the EhC2PK is present in the cytoplasm and phagocytosis cannot be initiated. This is followed by the recruitment of EhCaBP1 and actin. Overexpression of the C2 domain and the kinase-dead mutant of EhC2PK allowed formation of the initiation complex, but the process of phagosome formation was blocked; suggesting that progression of phagocytic cups to phagosomes requires additional steps, likely to involve the kinase domain of EhC2PK. As phagocytic cups did not form in cells overexpressing the kinase-dead mutant, it is likely that the kinase activity of EhC2PK may be needed for stabilization of the cups whose formation is initiated at the site of RBC attachment. We had earlier observed the presence of phagocytic cups but not phagosomes in cells overexpressing mutant CaBP1ΔEF, which can not bind Ca 2+ (ref. 31 ). Therefore, overexpression of the kinase-dead mutant form of EhC2PK and CaBP1ΔEF led to slightly different phenotypes and suggested that Ca 2+ signalling through EhCaBP1 may be required after participation of EhC2PK. These results show that the transition from initiation of phagocytosis to phagosome formation requires multiple steps, which include kinase reaction of EhC2PK and Ca 2+ -based signalling from EhCaBP1, apart from other factors described in the previous studies [7] . The absence of EhC2PK and EhCaBP1 from phagosomes is a clear indicator that their role is primarily in the process of initiation. The proposed mechanism also explains the process by which a predominantly cytoplasmic protein, EhCaBP1, accumulates at the membrane of the phagocytic cup. We are currently searching for additional molecules that may also be involved in the initiation steps. A number of C2-domain-containing proteins, such as PKCs, phospholipases and PI3K are known to participate in phagocytosis [37] , [38] , [39] . Though their role in phagosome closure is well documented, it is not clear whether these are also involved in the initiation. Phosphoinositides are also known to be important molecules in phagocytosis [39] . Inhibitors of PI3 kinase block erythrophagocytosis. In E. histolytica , these molecules participate mostly during the closing step of phagosome formation and not at the initiation step [26] . EhC2PK is different from all C2-domain-containing proteins that participate in phagocytosis. This is the first example of the direct participation of two Ca 2+ -binding proteins, EhC2PK and EhCaBP1, in the initiation of phagocytosis. Though there may be significant differences in the mechanisms of phagosome initiation in different organisms, and a variety of molecules may be involved in the process, it is likely that a similar theme may be operational in other systems. Moreover, phagocytosis is an essential process in many organisms including E. histolytica in which cellular proliferation is inhibited on blocking phagocytosis [30] . Unravelling the mechanism of phagocytosis may be helpful in finding novel targets for the development of new therapeutics. Growth and maintenance of parasites E. histolytica strain HM-1: IMSS and all transformed parasites were maintained and grown in TYI-S-33 medium containing 125 μl of 250 U ml −1 benzyl penicillin and 0.25 mg ml −1 streptomycin per 100 ml of medium [30] . The transformants containing tetracycline inducible system were grown in the presence of 10 μg ml −1 of hygromycin B. The cells were first grown for 48 h (60–70% confluent) and then 20 μg ml −1 tetracycline was added to the medium for 36 h for induction. Cells carrying constructs with constitutive expression system (such as GFP) were maintained at 10 μg ml −1 of G418. But the experiments were carried out in the presence of 30 μg ml −1 of G418. Transfection and selection of E. histolytica trophozoites Transfection was performed by electroporation. The trophozoites were collected from log phase cultures and washed with PBS followed by incomplete cytomix buffer (10 mM K 2 HPO 4 /KH 2 PO 4 (pH 7.6), 120 mM KCl, 0.15 mM CaCl 2 , 25 mM HEPES (pH 7.4), 2 mM EGTA, 5 mM MgCl 2 ). The washed cells were then re-suspended in 0.8 ml of complete cytomix buffer (incomplete cytomix containing 4 mM adenosine triphosphate, 10 mM glutathione) containing 200 mg of plasmid DNA and subjected to two consecutive pulses of 3,000 V cm −1 (1.2 kV) at 25 mF (Bio-Rad, electroporator). The transfectants were initially allowed to grow without any selection. Drug selection was initiated after 2 days of transfection in the presence of 10 μg ml −1 G418 for constructs with GFP or 10 μg ml −1 of hygromycin B was used for tetracycline inducible constructs. Cloning of various constructs used The CAT gene of the shuttle vector pEhHYG-tetR-O-CAT was excised using Kpn I and Bam HI and EhC2PK gene was inserted in its place in either the sense or the antisense orientation. Antisense and Sense forward and reverse primers used are shown in Supplementary Table S2 . The full-length gene was cloned in Bam H1 site in the case of GFP vector resulting in GFP tag on amino terminal of protein. Kinase domain was also cloned in constitutive (GFP) vector in Bam H1 site. The C2-GFP was made by introducing stop codon at 103 amino-acid residue by site-directed mutagenesis. Also K mutant was made by site-directed mutagenesis by changing 179th lysine to alanine. The sequences of oligonucleotides used for making the above stated constructs are described in Supplementary Table S2 . Immunoprecipitation from E. histolytica lysate Anti-EhC2PK antibody was conjugated to CNBr-activated Sepharose for immunoprecipitation. CNBr-activated Sepharose-4B (1 g, Pharmacia) was activated and processed as per the manufacturer's protocol. Briefly, crude immunoglobulins were collected from the immunized serum using 40% ammonium sulphate and subsequently dialysed in coupling buffer (bicarbonate buffer). Usually, 10 mg protein was added per gram of resin. The resin was mixed gently for 18 h at 4 °C. After coupling the coupled resin was processed as per manual provided by the manufacturer. The conjugated CNBr-Sepharose beads were incubated with E. histolytica lysate for 4 h at 4 °C. The beads were then washed with wash buffer (10 mM Tris-Cl (pH 7.5), 150 mM NaCl, 1 mM imidazol, 1 mM magnesium acetate, 2 mM β-ME and protease inhibitor cocktail) three times. The Ca 2+ and EGTA were maintained throughout the process as required. Beads were washed with 60 mM Tris-Cl (pH 6.8) and 100 mM NaCl. Finally, beads were washed with 60 mM Tris-Cl (pH 6.8). The pellet was suspended in 2× SDS polyacrylamide gel electrophoresis (PAGE) buffer and boiled for 5 min followed by centrifugation for 5 min. The proteins were then analysed by western blotting. Immunofluorescence staining E. histolytica cells were collected by centrifugation and washed before re-suspending in TYI-33 medium. The cells were then transferred onto acetone-cleaned coverslips placed in a petri dish and allowed to adhere for 10 min at 35.5 °C. The culture medium was removed and the cells were fixed with 3.7% pre-warmed paraformaldehyde for 30 min. After fixation, the cells were permeabilized with 0.1% Triton X-100/PBS for 1 min. The fixed cells were then washed with PBS and quenched for 30 min in PBS containing 50 mM NH 4 Cl. The coverslips were blocked with 1% BSA/PBS for 30 min, followed by incubation with primary antibody at 37 °C for 1 h. The coverslips were washed with PBS followed by 1% BSA/PBS before incubation with secondary antibody for 30 min at 37 °C. Antibody dilutions used were: anti-EhC2PK at 1:200, anti-EhCaBP1 at 1:200, anti-rabbit Alexa 488 and 556, anti-mice Alexa556 (Molecular Probes) at 1:300, TRITC-Phalloidin at 1:250. The preparations were further washed with PBS and mounted on a glass slide using DABCO (1,4-diazbicyclo (2,2,2) octane (Sigma) 2.5% in 80% glycerol). The edges of the coverslip were sealed with nail-paint to avoid drying. Confocal images were visualized using an Olympus Fluoview FV1000 laser scanning microscope. Erythrophagocytosis assay Ten million RBCs were washed with PBS and incomplete TYI-33. These were then incubated with 10 5 entamoeba for varying times at 37 °C in 0.5 ml of culture medium. The entamoebae and erythrocytes were centrifuged to get a pellet, non-engulfed RBCs were lysed with cold distilled water and re-centrifuged at 1,000 g for 2 min. This step was repeated twice, followed by re-suspension in 1 ml formic acid to lyse entamoebae containing engulfed RBCs. The absorbance was measured at 400 nm. Liposome-binding assay The liposomes were prepared as per protocol provided by Avanti Polar Lipid, Inc. http://avantilipids.com . The proteins were incubated with liposomes in binding buffer (Tris-Cl (pH 7.5) 10 mM, β-ME 0.25 mM, NaCl 50 mM). CaCl 2 was used at 2 mM wherever mentioned and EGTA was used at concentration of 5 mM at 37 °C for 2 h with intermittent tapping. The liposomes were centrifuged at 18,000 g for 30 min and subsequently washed with binding buffer to remove the nonspecific-binding proteins. Liposomes were than dissolved in SDS buffer and separated on SDS–PAGE and subsequently analysed for the presence of proteins by western analysis. For actin-binding assay the liposomes were incubated in polymerization buffer (Tris-Cl (pH 7.5) 10 mM, MgCl 2 20 mM, KCl 50 mM, ATP 2.5 mM, β-ME 2.5 mM) with EhC2PK, EhCaBP1 and actin. GST-bead pull down assay Purified GST-EhC2PK was incubated with Glutathione beads (Amersham) for 1 h at 4 °C in 1% PBS/BSA. Then EhCaBP1 or E. histolytica lysate as indicated was added to the reaction and incubated for 2 h at 4 °C. The beads were then washed with 1% PBS/BSA three times, and twice with PBS. Protein was eluted by adding 2× SDS–PAGE buffer followed by boiling for 5 min. The proteins were then analysed by western blotting. The same procedure was followed for other proteins with GST-tags. Western analysis For immunodetection, samples were separated on 8% SDS–PAGE. The gel was then transferred on to a polyvinylidine fluoride membrane and processed using standard methods. The antigens were detected with polyclonal antibodies raised in rabbit and mice followed by secondary anti-rabbit and anti-mice immunoglobulins conjugated to HRPO (1:10,000, Sigma). ECL reagents were used for visualization (Millipore). GFP and GST antibodies used were obtained from Molecular probes and Santa Cruz, respectively. The concentration of proteins in a sample was estimated by bicinchoninic acid assay using BSA as a standard. SDS–PAGE analysis was carried out in 10–12% acrylamide gels under reducing conditions according to the method of Laemmli. Statistical analysis Statistical comparisons were made using a one-way ANOVA test. Experimental values were reported as the means±s.e. Differences in mean values were considered significant at P <0.05. All calculations of statistical significance were made using the GraphPad InStat software package (GraphPad). How to cite this article: Somlata et al . A C2 domain protein kinase initiates phagocytosis in the protozoan parasite Entamoeba histolytica . Nat. Commun. 2:230 doi: 10.1038/ncomms1199 (2011).